Chemical influence on β-relaxations and the formation of molecule-like metallic glasses Secondary (also known as Johari-Goldstein or β-) relaxations are an intrinsic feature of supercooled liquids and glasses. They are important in many respects but the underlying mechanisms are not well understood. A long-standing puzzle is why some glasses show β-relaxations as pronounced peaks, whereas others as unobvious excess wings. Here we demonstrate that these different behaviours are related to the fluctuations of chemical interactions by using prototypical systems of metallic glasses. A general rule is summarized: pronounced β-relaxations are associated with systems where all the atomic pairs have large similar negative values of enthalpy of mixing, whereas positive or significant fluctuations in enthalpy of mixing suppress β-relaxations. The emerging physical picture is that strong and comparable interactions among all the constituting atoms maintain string-like atomic configurations for the excitations of β-events and can be considered as the formation of molecule-like metallic glasses. Supercooled liquids and glasses display diverse relaxation dynamics [1] , [2] , [3] , [4] , [5] , [6] . In addition to the primary (α-) relaxations that are responsible for the viscous flow, a kind of secondary relaxation, called Johari-Goldstein or β-relaxation [7] , [8] , [9] , often exists at high frequencies or low temperatures. Recent studies have demonstrated that β-relaxations are an intrinsic and universal feature of supercooled liquids and glasses [1] , [8] , [10] , and they are of significance to the understanding of many key issues in glassy physics and material sciences [1] , ranging from glass transition phenomenon [10] , [11] , [12] , [13] , diffusions [14] , [15] , [16] , [17] , physical aging [18] , [19] to mechanical properties [20] , [21] and mechanisms of plastic deformations [21] , [22] , [23] , as well as the stabilities and crystallization of glassy materials [24] , [25] , [26] . Despite their importance, the behaviour of β-relaxation themselves are not well understood, as they seem to be system dependent and even more complex than α-relaxations [1] , [5] . In some supercooled liquids and glasses, β-relaxations manifest as distinct peaks in dielectric or mechanical loss spectra. In some other systems, β-relaxations appear to be absent and, instead, excess contributions to the tails of α-relaxations show up [5] . These so-called excess wings have been observed in many systems without well-resolved peaks of β-relaxations. Historically, excess wings and peaks of β-relaxations were considered as two different phenomena and the corresponding materials were defined as type A- and B-glass formers, respectively [5] . Now it is commonly recognized they are similar in nature and excess wings are due to underlying β-relaxations [1] , [8] , [13] , [27] , [28] . However, a basic question remains unclear: why do some glasses exhibit pronounced peaks of β-relaxation, whereas others display excess wings? This question fundamentally connects to the structural origin of β-relaxations, which is also a long-standing unsolved question in glassy physics. As these two issues are interrelated, a thorough investigation of the former could provide deeper insights of the latter, and vice versa . On the other hand, to understand the dominating factors that govern the behaviours of β-relaxation are of practical importance. For example, polymers and MGs with pronounced β-relaxations at relatively low temperatures (for example, below or near room temperature) usually exhibit good ductility and they are favoured for mechanical applications [20] , [21] . However, for the pharmaceuticals industry, β-relaxations are sometimes undesired and should be suppressed as they cause the devitrification and destabilization of glassy medicines, which have better solubility and bioavailability than their crystalline counterparts [1] , [10] , [24] , [25] . MGs have recently received a lot of attention as model systems for studying β-relaxations because of their rich phenomenology in relaxation behaviours, simple atomic structures compared with other glasses (for example, polymers and molecular glasses) and widely tunable compositions [13] , [14] , [15] , [21] , [22] , [29] . However, it is noted that studying β-relaxations in MGs is much more difficult than that in molecular and polymer glasses [8] . In this work, by systematic scrutiny of the composition-dependent β-relaxations in several prototypical systems of MGs, we show a strong chemical effect on the behaviours of β-relaxation. A general rule is summarized, that is, the behaviours of β-relaxations are correlated to the fluctuations of the chemical interactions among the constituting atoms. Specifically, pronounced β-relaxations are always associated with MGs that all the atomic pairs have large similar negative values of enthalpy of mixing and the difference among these values should be small; however, positive enthalpy of mixing or a large difference in the enthalpy of mixing suppresses β-relaxations. We interpreted these findings in terms of recent theoretical ideas [30] , that string-like excitations are essential for β-events. The implications of this result for the understanding of structural origins of β-relaxations in MGs are discussed. The obtained insights provide a practical guideline for controlling β-relaxations in MGs and have implications for other type of glasses. 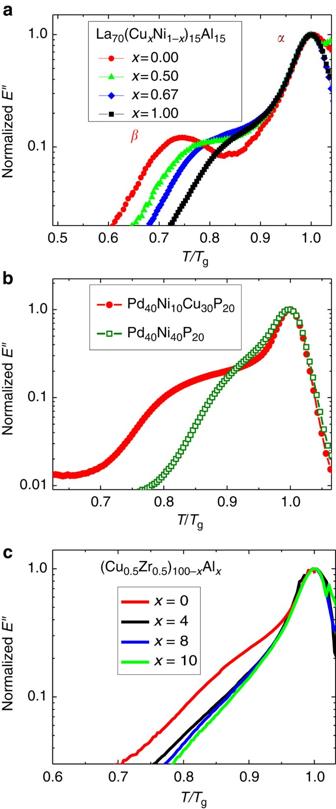Figure 1: Behaviours of β-relaxations in MGs. The normalized plot ofE′′as a function ofTgscaled temperature of (a) La70(CuxNi1−x)15Al15MGs with four differentxvalues as indicated; (b) Pd40Ni40P20and Pd40Ni10Cu30P20MGs; and (c) (Cu0.5Zr0.5)100−xAlxMGs with four differentxvalues as indicated. La-based MGs Figure 1a–c show the temperature T -dependent loss modulus E′′ (measured from dynamical mechanical analyser; see the Methods section) of the three MG systems in a normalized frame, where T and E′′ are scaled by the glass transition temperature T g and E′′ ( T = T g ), respectively. For clarity, curves only with testing frequency f =1 Hz are displayed. Figure 1a illustrates the effect of Cu substitution of Ni atoms on the behaviours of relaxation in the La 70 (Cu x Ni 1– x ) 15 Al 15 MGs. For the Cu-free La 70 Ni 15 Al 15 MG, besides the usual α-relaxation around T g , a pronounced E′′ peak is observed in the temperature range 0.6–0.8 T g , corresponding to the β-relaxation in the deep glassy state. With the increasing concentration of Cu to replace Ni atoms, the peaks of β-relaxation shift gradually to higher-scaled temperatures and become less pronounced. Eventually, β-relaxation in the Ni-free La 70 Cu 15 Al 15 MG manifests as a shallow shoulder on the low-temperature tail of α-relaxation. As Ni and Cu have nearly the same atomic sizes but different electron configurations (3d 8 4 s 2 and 3d 10 4 s 1 , respectively), the above result indicates a strong chemical effect on the behaviours of β-relaxations–in the La 70 (Cu x Ni 1− x ) 15 Al 15 MGs, Cu suppresses β-relaxations making them less pronounced, whereas Ni promotes them. Figure 1: Behaviours of β-relaxations in MGs. The normalized plot of E′′ as a function of T g scaled temperature of ( a ) La 70 (Cu x Ni 1− x ) 15 Al 15 MGs with four different x values as indicated; ( b ) Pd 40 Ni 40 P 20 and Pd 40 Ni 10 Cu 30 P 20 MGs; and ( c ) (Cu 0.5 Zr 0.5 ) 100− x Al x MGs with four different x values as indicated. Full size image Pd-based MGs The effect of Ni/Cu on the behaviours of β-relaxation in Pd 40 (Cu x Ni 1– x ) 40 P 20 MGs is presented in Fig. 1b . For the Cu-free Pd 40 Ni 40 P 20 MG, its β-relaxation manifests as a weak shoulder that superimposed on the tail of α-relaxation. Replacing Ni by Cu atoms in this system makes β-relaxations more pronounced and separated from α-relaxations (shift to lower-scaled temperatures). This observation demonstrates again a strong chemical effect on the behaviours of β-relaxation; however, in contrast to the La 70 (Cu x Ni 1– x ) 15 Al 15 system shown in Fig. 1a , Cu promotes β-relaxations in the Pd 40 (Cu x Ni 1– x ) 40 P 20 system. Such a comparison indicates the effect of Ni/Cu on the behaviours of β-relaxation is not solely determined by their atomic properties but dependent on their specific chemical environments and the interactions with other constituting atoms. This is different from some other properties of MGs. For example, the elastic modulus of MGs can be approximated by a simple ‘rule-of-mixture’ [31] and largely determined by the main constituting elements [32] . For the considerations of glass-forming ability, Ni and Cu are even sometimes regarded as same [33] , [34] . Distinctively, we note the mechanical behaviours (especially, the ductility and toughness) of MGs are sensitive to chemical effects [35] , [36] , in agreement with the notion that mechanical properties and β-relaxations are correlated [21] , [22] . CuZr-based MGs Fig. 1c shows the effects of Al alloying in a (Cu 0.5 Zr 0.5 ) 100– x Al x MG system. For the Al-free Cu 50 Zr 50 MG, its β-relaxation manifests a weak but discernable shoulder, whereas a minute mount of Al alloying (about 4%) drastically suppresses the shoulder and an excess wing shows up instead. With further alloying of Al, the excess wings persist and become more closely merged with α-relaxations. This result demonstrates microalloying has important influence on the behaviours of β-relaxation as well. All these findings above demonstrate a strong and complicated (system specific) chemical effect on the behaviours of β-relaxation in MGs. A pertinent question is how to understand these system-specific behaviours in a general physical scenario. To appreciate this question, we consider the concept of enthalpy of mixing for MGs as it provides an effective way to the understanding of many chemical-related issues in MGs, such as glass-forming ability [33] , [34] , mechanical properties [37] , phase separation [38] , [39] , [40] , as well as crystallization and devitrification of MGs [41] . Fig. 2a–c display the values of enthalpy of mixing , for different atomic pairs in these three prototypical MG systems [34] . They are obtained from Miedema’s model for binary alloys (with equiatomic composition, A 50 B 50 ) [34] , [42] , which is a semi-quantitative theory based on the thermodynamics of materials and energy band theory. We first evaluated the mean chemical affinity Δ H chem for these MGs. As suggested in Takeuchi et al . [34] and He et al . [35] , the Δ H chem of a given multicomponents alloy can be estimated using a weighted average approach, (where c A and c B are the molar percentage of the elements A and B, respectively). 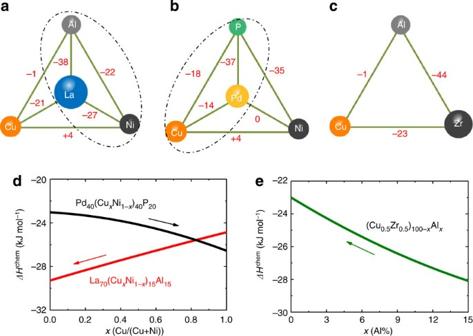Figure 2: Enthalpy of mixing and mean chemical affinity of MGs. The enthalpy of mixing for the constituting atomic pairs in (a) La-Ni-Cu-Al (b) Pd-Ni-Cu-P and (c) Zr-Cu-Al systems; and the compositional-dependent mean chemical affinity ΔHchemfor (d) La70(CuxNi1−x)15Al15and Pd40(CuxNi1−x)40P20MGs and (e) (Cu0.5Zr0.5)100−xAlxMGs. The units ina–care kJ mol−1. Dash-dot ellipses ina,bindicate compositions with pronounced β-relaxations; arrows ind,eindicate the directions along which β-relaxations become more pronounced with composition variations in each systems. Figure 2d shows the Δ H chem as a function of x =(Cu/(Cu+Ni)) for the La 70 (Cu x Ni 1- x ) 15 Al 15 and Pd 40 (Cu x Ni 1– x ) 40 P 20 MG-systems. It is observed all the compositions in both systems have large negative values of Δ H chem in the range of −20 to −30 kJ mol −1 . The largest negative values of Δ H chem are found at composition points of La 70 Ni 15 Al 15 and Pd 40 Cu 40 P 20 for the two systems, respectively, and interestingly both of the compositions show pronounced β-relaxations. The dependence of Δ H chem against x is also correlated with the compositional-dependent behaviours of β-relaxation in these two systems, which seems to indicate a trend that the larger negative values of Δ H chem the more pronounced β-relaxations. However, we find this observation is not applicable to the (Cu 0.5 Zr 0.5 ) 100– x Al x systems. As shown in Fig. 2e with microalloying of Al, the Δ H chem becomes more negative but β-relaxation becomes less pronounced (cf. Fig. 1c ), which is opposite to the expectation from that of La 70 (Cu x Ni 1– x ) 15 Al 15 or Pd 40 (Cu x Ni 1– x ) 40 P 20 . These results imply (i) large negative values of Δ H chem might be a necessary condition but not sufficient to guarantee pronounced β-relaxations; (ii) although the correlation between Δ H chem and the behaviours of β-relaxation are interesting and useful for the La- and Pd-based MGs, it is system specific and thus not universal (at least not suitable for Cu-Zr-Al MGs); (iii) and there must be other underlying influential factors that govern the behaviours of β-relaxation beyond the ‘mean-field’-like approach to the mean chemical affinity. Figure 2: Enthalpy of mixing and mean chemical affinity of MGs. The enthalpy of mixing for the constituting atomic pairs in ( a ) La-Ni-Cu-Al ( b ) Pd-Ni-Cu-P and ( c ) Zr-Cu-Al systems; and the compositional-dependent mean chemical affinity Δ H chem for ( d ) La 70 (Cu x Ni 1− x ) 15 Al 15 and Pd 40 (Cu x Ni 1− x ) 40 P 20 MGs and ( e ) (Cu 0.5 Zr 0.5 ) 100− x Al x MGs. The units in a – c are kJ mol −1 . Dash-dot ellipses in a , b indicate compositions with pronounced β-relaxations; arrows in d , e indicate the directions along which β-relaxations become more pronounced with composition variations in each systems. Full size image We next take into account of the fluctuations of chemical interactions. A closer examination of for these different atomic pairs shown in Fig. 2a–c reveals the following clue. In systems with pronounced β-relaxations, all the atomic pairs have large negative and comparable values of , whereas systems with positive enthalpy of mixing or large difference in the enthalpy of mixing are associated with less pronounced β-relaxations or excess wings. For instance, in the La-Ni-Al system with pronounced β-relaxations, the for La-Ni, La-Al and Ni-Al atomic pairs are −28, −37 and −22 kJ mol −1 , respectively, whereas in the La-Cu-Al system with less pronounced β-relaxations, for Al-Cu is −1 kJ mol −1 , much smaller than that for other two atomic pairs (−21 and −37 kJ mol −1 for La-Cu and La-Al atomic pairs, respectively), and thus there is a large difference in enthalpy of mixing between different atomic pairs. This finding is also applicable to Pd-Cu/Ni-P and Zr-Cu-Al systems as shown in Fig. 2b,c respectively. We have verified that above finding also holds in other 12 ternary MG systems (see Table 1 ), including RE-TM-Al (where RE=La, Pr, Nd, Sm, Gd and Er; TM=Co, Ni and Cu; their β-relaxations are pronounced peaks for TM=Co and Ni and shoulders for TM=Cu), Zr-Cu-Ag (excess wings), Cu-Ti/Zr-Be (excess wings), Pt-Cu/Ni-P (humps) and Pd-Cu-Si (humps). One exception is observed in La/Ce-Cu-Al systems [8] , [43] where La-Cu-Al MGs have shoulder-like β-relaxations, whereas in Ce-Cu-Al MGs excess wings even La and Ce have the similar values of enthalpy of mixing with Cu and Al. This may be explained by the different electronic structures between La and Ce that are not accounted by the enthalpy of mixing from Miedema’s model. As the Miedema’s model is only empirical estimates, to obtain accurate values of enthalpy of mixing in a particular system, experiments or first-principle calculations are required. Besides, the values of enthalpy of mixing might even be concentration dependent. Furthermore, we caution that the approach of enthalpy of mixing does not consider the interactions between the same kinds of atoms, which could be important for binary or monatomic systems and systems with high concentrations of solvent atoms. Nevertheless, as the above systems are different in many respects and cover most of the known MGs, our findings thus indicate that both of the magnitude and fluctuations of chemical interactions among constituting atoms are influential factors to the behaviours of β-relaxation in MGs. Specifically, strong and comparable interactions among all the constituting atoms, which might be viewed as the local formation of molecule-like structures, are favourable for pronounced β-relaxations, otherwise for excess wings. These findings are compatible with a coupling model [1] , [9] , which suggests stronger interactions are beneficial for pronounced β-relaxations. Table 1 β -relaxation characteristics and enthalpy of mixing. Full size table Recently, a theoretical work predicts β-relaxation is related to the excitations of string-like configurations [30] , and a subsequent molecular dynamics simulation corroborated it [44] . Accordingly, a β-event is considered as a chain of atoms that moves back-and-forth reversibly and cooperatively within the confinement of surrounding elastic matrix [14] , [45] . In light of this scenario, it is reasonable that strong and comparable magnitudes of interactions among all the constituting atoms are necessary for archiving a critical length for the string-like atomic configurations for the movements of β–events, whereas weak interactions (or large fluctuations) between certain atomic pairs would break the string-like configurations, making them less cooperative. Presumably, weakly bonded atoms diffuse readily, and thus acting as ‘cutters’ or ‘anti-glue’ to the string. In other words, we suggest strong interactions hold neighbouring atoms together to form the string-like configurations and to complete cooperative β-events. We noted that maintaining a certain length of atomic/molecular chains has been inferred critical to the behaviours of β-relaxations in different types of glasses. For example, Mattsson et al . [46] studied the chain length-dependent relaxations in a series CH 3 O-[CH 2 CH(CH 3 )O] n -CH 3 organic glasses. By varying the chain length n =1, 2, 3 and ≈7 and in a polymer ( n ≈69), they found in dielectric spectra for n ≤3 β-relaxations manifest as excess wings, whereas a broad hump for n ≈7, and a distinct peak for the polymer ( n ≈69). A similar result was observed in polyalcohols by Döß et al . [47] These findings suggest that shortening the chain structures could suppress β-relaxations (other possible reasons are also noted in Ngai et al . [48] ). In Pd-Ni-Cu-P MG systems, several studies from the electronic and atomic structural perspectives have uncovered that with the increasing of Cu contents, the MGs acquire deeper binding energy and develop more covalent-like bonding, and especially chain-like Pd-P-Pd/Cu atomic configuration was suggested [49] , [50] , [51] . These findings are consistent with our observation that Cu promotes β-relaxations in Pd-Ni/Cu-P systems because of its strong interactions with Pd and P. In a Pd-Cu-Si MG, Bedorf and Samwer [45] studied the length-scale effects on relaxations and they found that by reducing the film thickness <30 nm, the β-relaxations are effectively suppressed. This result was explained because of the breakdown of the stress field surrounding the string-like excitation when free surfaces are reached and the pinning effects of free surface [45] . More recently, Casalini et al . [52] used -SCH 3 to replace -OCH 3 group in poly(methyl methacrylate) and they found in dielectric spectra that the intensity of the β-relaxation is substantially reduced, as the result of the electronegativity of sulphur is much less than that of oxygen [52] . Their observations demonstrated that tuning the chemical interactions can result in different behaviours of β-relaxation in polymers, similar with our findings in MGs. These results, together with our present findings, seem to suggest string-like motions of molecule-like structures are a universal mechanism of β-relaxation in glassy materials, ranging from MGs, molecular and polymer glasses. In summary, we identified an influential chemical effect on the behaviours of β-relaxations in MGs–large similar negative enthalpy of mixing among all the constituting atoms results in pronounced β-relaxation peaks in mechanical loss spectra, whereas positive or large fluctuations in the values of enthalpy of mixing suppress β-relaxations and usually associate with excess wings. The behaviour of β-relaxations is proposed to correlate with a characteristic length scale of string configurations. Our findings provide a practical guideline in controlling the behaviour of β-relaxations in MGs and have implications for other type of glasses as well. Sample preparation Three typical MG systems with 10 different compositions were selected for experiments; these are La 70 (Cu x Ni 1– x ) 15 Al 15 with x =0, 0.5, 0.67 and 1; Pd 40 (Cu x Ni 1– x ) 40 P 20 with x =0 and 0.75; and (Cu 0.5 Zr 0.5 ) 100– x Al x with x =0, 4, 8 and 10, respectively; because of their markedly different relaxation behaviours that are representative for most known MGs. The La-based and CuZr-based MGs are prepared by Cu-mold casting method: the raw materials were melted in a Ti-gettered argon atmosphere and subsequently cast into a water-cooled Cu-mold. The Pd-based MGs (with P containing) were prepared by induction melting of the raw materials in argon-filled and sealed quartz tube, additional B 2 O 3 were used as fluxing medium. The fluxed alloys were then re-melted and cast by Cu-mold casting method. Characterization The glassy nature of the samples was ascertained by X-ray diffraction (a MAC Mo3 XHF diffractometer with Cu K α radiation and a Bruker D8 with Cu Kα radiation) and differential scanning calorimeter (PerkinElmer DSC-7 and DSC-5). The dynamical mechanical spectroscopies of these MGs were measured on a TA Q800 dynamical mechanical analyser by single-cantilever bending method with a heating rate of 2 K min −1 , strain amplitude about 0.1% and discrete testing frequency of 1, 2, 4, 8, 16 and 32 Hz. How to cite this article: Yu, H. B. et al . Chemical influence on β-relaxations and the formation of molecule-like metallic glasses. Nat. Commun. 4:2204 doi: 10.1038/ncomms3204 (2013).